Chemical control over the energy-level alignment in a two-terminal junction The energy-level alignment of molecular transistors can be controlled by external gating to move molecular orbitals with respect to the Fermi levels of the source and drain electrodes. Two-terminal molecular tunnelling junctions, however, lack a gate electrode and suffer from Fermi-level pinning, making it difficult to control the energy-level alignment of the system. Here we report an enhancement of 2 orders of magnitude of the tunnelling current in a two-terminal junction via chemical molecular orbital control, changing chemically the molecular component between a stable radical and its non-radical form without altering the supramolecular structure of the junction. Our findings demonstrate that the energy-level alignment in self-assembled monolayer-based junctions can be regulated by purely chemical modifications, which seems an attractive alternative to control the electrical properties of two-terminal junctions. The possibility to integrate functional molecules into electronic devices is one of the promising approaches to miniaturize electronic circuits or to generate electronic function that is difficult to obtain using conventional semiconductors [1] , [2] , [3] . The advantage of molecular-based devices is, in principle, that the conductance can be tuned by designing molecules with the electronic and chemical structure tailored for the desired application. To achieve this ‘chemical control’ over transport characteristics, a good control over the energy-level alignment of the molecular frontier orbitals with respect to the Fermi level ( E F ) of the electrodes is needed. For instance, control over the energy-level alignment has been used in thin film devices to lower charge injection barriers by either altering the work function of the metal-electrodes [4] , or controlling the HOMO (highest-occupied molecular orbital) and/or LUMO (lowest unoccupied molecular orbital) levels with respect to the Fermi levels by chemical modification [5] , [6] , or introducing charge injection layers [7] , [8] . In practical systems, however, chemical control over the energy-level alignment proves to be challenging because of the so-called ‘pillow effect’ or Fermi-level pinning [7] . In molecular electronics, especially in the case of two-terminal devices, it remains difficult to predict how, if at all, certain chemical functionalities alter the junction characteristics [9] , [10] , [11] , [12] , [13] , [14] , [15] . Here we show how the tunnelling rates across molecular junctions can be increased by 2 orders of magnitude by tuning the energy levels of the system within the conduction window without the need for altering the molecular structure of the molecule–electrode interfaces by modifying the electronic structure of the molecules between the open- and closed-shell forms. Since the nature of the molecule–electrode interface is kept the same for both molecular forms, this approach is not limited by Fermi-level pinning. The molecule bridging the two electrodes provides the molecular energy levels ( E ) in the solid-state device for conduction channels. The sum of the channels ( M ( E )) within the electrochemical potential window between μ L and μ R , will result in an effective current, as described by the Landauer formalism [16] , [17] , [18] : where h is Planck’s constant, q is the electron charge and T ( E ) is the transmission probability, which is inversely proportional to the square of zero-bias energy off-set between the molecular orbital and the Fermi level of the electrodes (δ E ME ), equation (2), where Γ L and Γ R are the degree of the coupling strength between the molecular frontier orbital and the Fermi level of the left (L) and the right (R) electrodes, respectively. Thus, the current ( I ) is proportional to the M ( E ) and inversely proportional to (δ E ME ) (ref. 2 ). Although in three-terminal devices the energy-level alignment of the systems, that is, the value of δ E ME , can be controlled via a gate electrode (or in a wet electrochemical environment gating via the electrolyte is possible) [19] , [20] , [21] , [22] , in two-terminal devices, however, the molecular orbitals cannot be gated and therefore alternative approaches are needed. One of these approaches is to control the energy-level alignment of the system by modifying the chemical structure of the molecules inside the junctions. In reality, it is difficult to predict how changes to the chemical structure of the junctions affect the electrical properties of the junctions and seemingly contradicting results have been reported. In SAM-based junctions, the difficulty of controlling the energy-level alignment due to Fermi-level pinning has been well-recognized. [7] , [23] For example, Frisbie and co-workers [24] showed that changing the work function of the metal had a noticeable effect on the contact resistance (due to a large surface dipole at the metal–thiolate interface) but not on the energy-level alignment. Similarly, Blom and co-workers [25] found that introducing additional dipoles in the SAM structure results in large work function shifts. In contrast, Whitesides and co-workers [13] , [14] , [15] observed that the tunnelling rates across aliphatic SAMs in EGaIn junctions were independent of dipoles or acidity of small end groups of alkanethiolate SAMs. We confirmed these findings by Whitesides and co-workers [15] for a small subset of SAM structures, but Whitesides and co-workers and we also showed that other functionalities, such ferrocene (Fc) and redox-active aromatic groups [26] , [27] , [28] , or polarizable groups (halogens) [29] , did change the junction characteristics and induced rectification or changed the tunnelling rates, respectively. These studies show, as a group, that it is indeed difficult to predict which kind of chemical functionalities result in a noticeable change in the electrical characteristics of the junctions. One of the reasons is that changes in the molecular structure also result in changes of the molecule–electrode interactions and the supramolecular structure of the SAM making it difficult to isolate the factors that dominate the charge transport rates. In this study, the charge transport rate across SAM-based tunnelling junctions with the same electrode–molecule interfaces and supramolecular structure but with different electronic structure modified by chemically switching the molecule between the open- and closed-shell forms is investigated. In particular, we incorporate SAMs of polychlorotriphenylmethyl radical (PTM R ) and of non-radical polychlorotriphenylmethane (PTM NR ) molecules tethered to the Au bottom electrode via an alkanethiolate linker into EGaIn junctions. The open-shell form contains a SOMO (single occupied molecular orbital), with one electron with an α spin configuration, and a SUMO (single unoccupied molecular orbital), and this results in a smaller molecular energy SOMO–SUMO gap than the HOMO–LUMO gap of the closed-shell form (Δ E values in Fig. 1 ). Similar observations have been made in an organic thin film in a wet electrochemical environment [25] . Thus, we change the electronic structure of the PTM while keeping the PTM—electrode interactions the same as the PTM is separated from the top-electrode via a van der Waals interface and the bottom-electrode via the alkyl group. Moreover, we show that not only the energy gap is lowered but also the value of δ E ME (or in other words, the energy-level alignment changed) which results in a low tunnelling barrier height and thereby a high-tunnelling current. 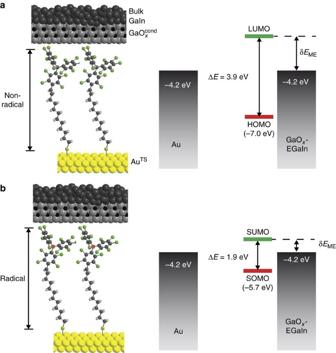Figure 1: Schematic illustrations of the junctions. Schematic representations of the junctions of AuTS-SC10PTMR/NR//GaOxcond/EGaIn and the corresponding energy level diagrams. The top-electrodes (a) are liquid metal GaOxcond/EGaIn (where EGaIn is the eutectic alloy of Ga and In, and GaOxcondis a 0.7-nm-thick self-limiting highly conductive oxide layer)15,16,17. The bottom electrodes (b) are template-stripped Au surfaces (∼300-nm-thick, see fabrication methods in ref.11and Methods for details). The ΔEand δEMErepresent the molecular energy gap and zero-bias energy off-set between the LUMO (or SUMO) and the Fermi level of the electrodes, respectively. Red dots show the central C atoms of radical moieties. The distance (d) between two electrodes is about 2.1 nm. Figure 1: Schematic illustrations of the junctions. Schematic representations of the junctions of Au TS -SC 10 PTM R/NR //GaO x cond /EGaIn and the corresponding energy level diagrams. The top-electrodes ( a ) are liquid metal GaO x cond /EGaIn (where EGaIn is the eutectic alloy of Ga and In, and GaO x cond is a 0.7-nm-thick self-limiting highly conductive oxide layer) [15] , [16] , [17] . The bottom electrodes ( b ) are template-stripped Au surfaces ( ∼ 300-nm-thick, see fabrication methods in ref. 11 and Methods for details). The Δ E and δ E ME represent the molecular energy gap and zero-bias energy off-set between the LUMO (or SUMO) and the Fermi level of the electrodes, respectively. Red dots show the central C atoms of radical moieties. The distance ( d ) between two electrodes is about 2.1 nm. Full size image We investigated the mechanism of charge transport through a SAM of a free organic radical based on PTM radical because it is stable and can be readily grafted on gold [30] , [31] , glass [32] and ITO [33] , or as a single molecule linked between gold electrodes showing a Kondo effect at low temperatures [34] . The PTM radical has one unpaired electron located on the central carbon atom with a sp [2] hybridization, which is structurally shielded by the bulky o -chlorine atoms, leading to a high chemical and thermal stability [35] . This radical can be readily converted to the alpha-H non-radical derivative via reduction to the anion and protonation of the central carbon. Previously, the charge transport rates across PTM R/NR SAMs on gold were investigated by conductive probe atomic force microscopy (cpAFM), showing a higher tunnelling rate across junctions with PTM R -based SAMs than those junctions with PTM NR -based SAMs [36] , [37] . Theoretical calculations of the electronic structure of the gas phase molecules suggested SUMO-assisted transport in the case of the radical-based SAM. Based on these calculations, it was assumed that the mechanism of charge transport was coherent tunnelling without direct experimental evidence regarding the electronic structure of the junction- or temperature-dependent charge transport data. This assumption, however, may have been not correct because in these studies the PTM moiety was grafted to the bottom-electrode via a short-conjugated tether. Likely significant hybridization of the molecular frontier orbital with the gold electrode occurs and resonant transport cannot be excluded. Here we demonstrate that the mechanism of charge transport is coherent tunnelling in both types of PTM R/NR SAMs bearing long (6 or more CH 2 units) non-conjugated alkyl tether, to ensure the molecular frontier orbitals remain localized on the PTM and that tunnelling rates across the junction can be increased by 2 orders of magnitude in the open-shell based SAMs with respect to the closed-shell ones without changing the tunnelling distance d or the nature of the molecule–electrode contacts. This increase in the tunnelling rates is because in junctions with the PTM R SAMs, the SUMO participates in the transport and effectively lowers the tunnelling barrier height (see Fig. 1 ). Importantly, contrary to what we hypothesized in previous works [36] , [37] , the findings reported here unambiguously demonstrate that the enhancement of the tunnelling rate transport across the radical-based SAMs is not due to a resonant tunnelling mechanism but instead due to a SUMO-assisted coherent non-resonant tunnelling. We base our conclusions on statistically large numbers of J (V) data and J (V,T) measurements combined with a detailed physical-organic study of the electronic and supramolecular SAM structures using six newly designed PTM derivatives with different chain lengths. All SAMs are anchored on gold via a thiolate binding group and the PTM R/NR moieties are effectively decoupled from the electrode via the long alkyl chains. Hence, all types of SAMs yield similar work functions of gold. Here we show intramolecular control over the electronic structure of the junction, resulting in a large change in the value of δ E ME and, consequently, the observed tunnelling rates. In other words, we show a large modulation of the tunnelling rate of 2 orders of magnitude across junctions with the same supramolecular structure and work function of the electrodes. Molecular synthesis Three PTM-CH=CH-(CH 2 ) n −2 SH radicals and three αH-PTM-CH=CH-(CH 2 ) n −2 SH non-radicals, with n =8, 10 and 12, have been synthesized. We use the abbreviations HSC n PTM R/NR for simplicity to follow the discussions. 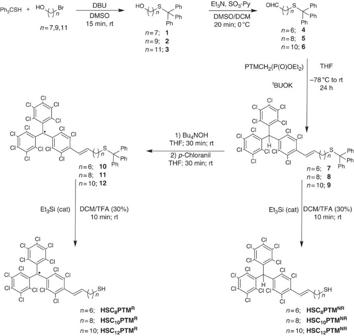Figure 2: Synthetic route to radicals HSCnPTMRand non-radicals HSCnPTMNR. DBU, 1, 8-diazabicycloundec-7-ene;tBuOK, potasium tert-butoxide; DMSO, dimtehylsulfoxide; DCM, dichloromethane; ET3N, triethylamine; SO3Py, sulfur trioxide pyridine; Bu4NOH, tetrabutylammonium hydroxide; ET3Si, triethylsilane; THF, tetrahydrofurane; TFA, trifluoroacetic acid; rt, room temperature. Figure 2 shows the synthetic route to the PTM-thiolated derivatives HSC n PTM R/NR . We aimed to couple the alkyl chain with the thiol-anchoring group to the PTM unit using a C=C bond, because the double bond only causes a small modification to the electronic structure of the PTM (unlike electron donating/withdrawing groups such as amides or carbonyls) and it can be readily formed by a Wittig–Horner reaction between the PTM-phosphonate and an aldehyde bearing the corresponding alkyl chain and the thiol-precursor [38] . To overcome the instability of the thiol groups under the Wittig–Horner conditions, as well as under the oxidative conditions needed to generate the radical from the corresponding carbanion, we used a triphenylmethyl (trityl) as a protecting group. This protecting group was easily deprotected in acidic media in the last step of the synthesis to obtain the final thiolated compounds ( Fig. 2 ). High-pressure liquid chromatography (HPLC) confirmed that, despite the reducing character of the thiol groups and the low-reduction potential of the PTM radicals [21] , PTM-thiolated derivatives are stable for several weeks in ambient conditions. We note that storing for extended periods of time disulfide derivatives formed as a result of the oxidation of the thiol groups. The same was observed for the non-radical counterparts and, for this reason, all SAMs reported here were prepared using freshly deprotected thiolate derivatives. Figure 2: Synthetic route to radicals HSC n PTM R and non-radicals HSC n PTM NR . DBU, 1, 8-diazabicycloundec-7-ene; t BuOK, potasium tert-butoxide; DMSO, dimtehylsulfoxide; DCM, dichloromethane; ET 3 N, triethylamine; SO 3 Py, sulfur trioxide pyridine; Bu 4 NOH, tetrabutylammonium hydroxide; ET 3 Si, triethylsilane; THF, tetrahydrofurane; TFA, trifluoroacetic acid; rt, room temperature. Full size image SAM structural characterization The SAMs were prepared using freshly template-stripped Au surfaces with ultra-flat topography [39] , [40] , [41] , which were immersed in 0.5 mM solutions of the target compound in toluene. Before the fabrication of the top-electrode, the SAMs were characterized by cyclic voltammetry (CV) and angle-resolved X-ray photoelectron spectroscopy (ARXPS) to ensure that we used good-quality SAMs (See Supplementary Fig. 10 and Supplementary Figs 13–16 for the complete data sets). The ARXPS and element ratios (see more details in Method section ‘Photoelectron spectroscopy’ and ‘Determination of the thickness of the SAMs from the S 2 p spectra’) analysis from XPS revealed that both radical and non-radical SAMs are in a standing-up phase rather than lying flat on the surface, the calculated layer thickness ( d ) scales with n and was similar for PTM NR and PTM R SAMs with the same number of n , and that all SAMs had very similar surface coverage (1.4–1.6 × 10 −9 mol cm −2 ) within experimental error (5%) (see Supplementary Table 1 and Methods ). From our results, we conclude that the supramolecular structure of the SAM does not change when the PTM units are in the open- or closed-shell forms. SAM electronic structure characterization The electronic structure of the SAMs on Au TS was determined by ultraviolet photoelectron spectroscopy (UPS) and near edge X-ray adsorption fine structure spectroscopy (NEXAFS) to estimate the positions of the filled and empty states, respectively. The UPS spectra were recorded to determine their energy levels with respect to the Fermi level of a clean Au substrate for all PTM R/NR -Au TS SAMs. 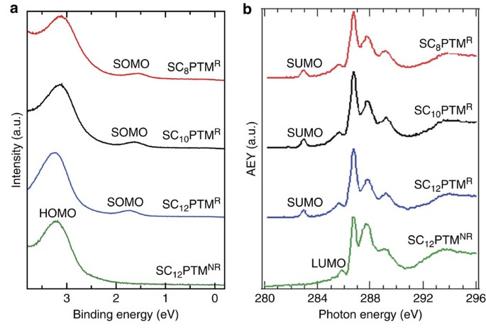Figure 3: Electronic structure of the PTMR/NRSAMs on AuTS. (a) Ultraviolet photoemission spectroscopy (UPS) and (b) C K-edge X-ray absorption fine structure (NEXAFS) spectra of SAMs derived from HSCnPTMRwithn=8, 10, 12 and HSC12PTMNR. Figure 3a shows the UPS spectra of the HSC n PTM R SAMs. We found that the SOMO peak with a SOMO-onset value of ∼ 1.45 eV is clearly visible in contrast to the spectra obtained from HSC n PTM NR SAM that do not show this peak (here only HSC 12 PTM NR SAM is shown as representative of the PTM NR SAMs; see Supplementary Fig. 17 for n =8 and 10) and only reveal the HOMO peak with the HOMO-onset value at ∼ 2.45 eV. This is a clear evidence of the persistence of the unpaired electron once the molecules are covalently grafted on the surface. Figure 3: Electronic structure of the PTM R/NR SAMs on Au TS . ( a ) Ultraviolet photoemission spectroscopy (UPS) and ( b ) C K-edge X-ray absorption fine structure (NEXAFS) spectra of SAMs derived from HSC n PTM R with n =8, 10, 12 and HSC 12 PTM NR . Full size image The C K-edge NEXAFS spectra ( Fig. 3b ) show peaks at ∼ 285.7 and ∼ 286.5 eV, which are assigned to the C(Ph)→ π * transitions in the perchlorinated phenyl rings of the PTM molecules [42] . These peaks are present in the spectra of PTM R and PTM NR SAMs, but in the case of the PTM R SAMs there is an additional peak at ∼ 282.9 eV. This peak indicates the presence of an empty state with an energy just above the Fermi level and it is attributed to the transition to the SUMO orbital [42] , [43] . We have calculated the SUMO (for the PTM R SAMs) and LUMO (for the PTM NR SAMs) energy position from the NEXAFS spectra ( Table 1 , see details in Methods). Thus, the molecular energy gap of the PTM R/NR SAMs could be calculated from UPS and NEXAFS spectra ( Table 1 ) and the results are comparable with the optical band gap ( ∼ 1.9 eV for R and ∼ 3.9 eV for NR) determined by the ultraviolet–visible spectra (see Supplementary Figs 6 and 7 ). Table 1 Statistics of electrical characterization of the PTM-based junctions and energy level determination by UPS and NEXAFS spectroscopy at room temperature. Full size table We note that the energy levels determined by these techniques only involve SAMs. We believe that the energy levels shift once the SAMs form a contact with the GaO x cond /EGaIn top-electrodes, though we believe these shifts are small due to the non-covalent nature of the SAM//GaO x cond /EGaIn contact. Thus, the energy levels depicted in Fig. 1 give a good qualitative indication of the energy levels. Moreover these experimental data indicate that the SUMOs of radical and LUMOs of non-radical SAMs, are closer to the E F of GaO x /EGaIn (−4.2 eV) [44] and SAM-modified Au TS bottom electrodes (−4.1 to −4.2 eV) than the SOMO and HOMO. Therefore we believe the mechanism of charge transport involves tunnelling via the SUMO or LUMO orbitals. We note that the nature of the charge carrier cannot be directly measured in these two-terminal devices, but our results agree with the findings reported by Cahen and co-workers [45] for n -alkanethiolate SAMs that showed that transport is dominated by the unoccupied molecular orbitals. Transport through the SAMs For this study, we used liquid metal GaO x cond /EGaIn top-electrodes since they form non-invasive soft top-contacts with the SAMs [11] , [46] , [47] . To fabricate the molecular junctions, the HSC n PTM R/NR derivatives were first self-assembled on ultra-smooth Au TS bottom electrodes and followed by the formation of the top-electrodes following previously reported methods (see Methods) [48] , [49] . The Au TS -SC n PTM R/NR //GaO x cond /EGaIn junctions were measured under the same experimental conditions and we biased the top-electrodes and grounded the bottom electrodes. We collected at least 21 traces on 20 different junctions for each type of junctions (see Table 1 for all statistics). The data were plotted in histograms of log 10 | J | at each applied bias (voltage steps of 0.05 V), and then we fitted Gaussians to the histograms to obtain the mean values of log 10 | J | ( ‖ J ‖ > G ), log-s.d. ( σ log ) and 95% confidence intervals. 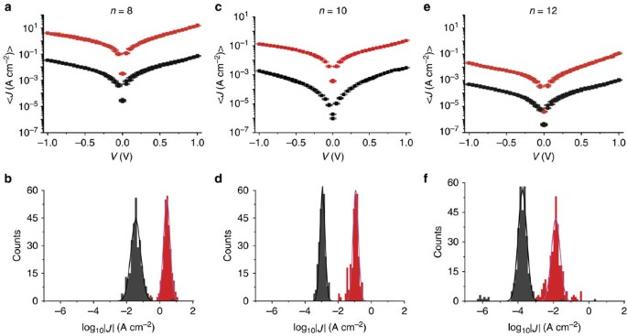Figure 4: Electrical characteristics of the tunnelling junctions at room temperature. (a,c,e) Plots of the‖J‖>Gagainst the applied bias for radical (red) and non-radical (black) junctions and (b,d,f) the histograms of log‖J‖measured at −1.0 V along with Gaussian fits to these histograms. Figure 4 shows ‖ J ‖ > G plotted against the applied bias with 95% confidence levels as error bars of the junctions and the histograms of log 10 | J | at –1.0 V for the PTM R/NR SAMs (red corresponds to the radical and black to the alpha-H non-radical SAMs). In all cases, the values of ‖ J ‖ > G measured for the PTM radical SAMs are consistently about 100 times higher than those values obtained for junctions with the non-radical SAMs in the whole measured bias range. The higher measured current across the radical SAMs is in agreement with our previous studies involving junctions based on cpAFM and electron transfer rate studies of different types of PTM-based SAMs [36] , [37] . Figure 4a also shows that ‖ J ‖ > G values at +1.0 V are ∼ 1.5 times higher than at −1.0 V; this small asymmetry in the J (V) curves could be caused by the different electrode materials, different interfaces at top- and bottom-contact, or the negative dipole moment of the PTM molecules due to electron-withdrawing character of chlorinated phenyl rings [30] , [50] . Figure 4: Electrical characteristics of the tunnelling junctions at room temperature. ( a , c , e ) Plots of the ‖ J ‖ > G against the applied bias for radical (red) and non-radical (black) junctions and ( b , d , f ) the histograms of log ‖ J ‖ measured at −1.0 V along with Gaussian fits to these histograms. Full size image To investigate the charge transport mechanism in more detail, we carried out temperature-dependent charge transport measurements in the range of temperatures ( T ) from 340 to 210 K. We used a device made of a polymeric transparent polydimethylsiloxane (PDMS) mold having micro-channels that stabilize the GaO x cond /EGaIn (see ref. 51 and Methods for details). The GaO x cond /EGaIn formed contact with the SAM through small round-orifices present in the polymeric mold. These devices generate stable junctions over at least 1,000 traces (see Supplementary Fig. 12 ) and allow us to perform temperature-dependent measurements in the probestation. 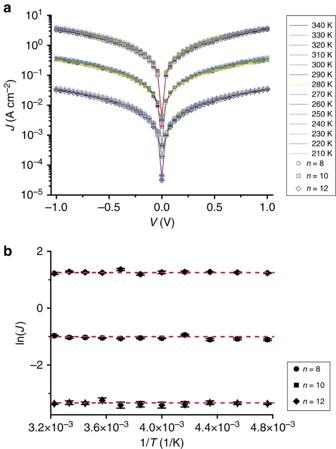Figure 5: Temperature dependence measurements. (a) Semi-log plots of the averageJ(V) curves measured over the temperature range of 210–340 K at intervals of 10 K for AuTS-SCnPTMRSAMs withn=8, 10 and 12 and (b) Arrhenius plots of the averageJat −1.0 V. The error bars represent the standard deviations of 10J(V) curves. Figure 5a shows averaged J (V) curves from 10 J (V) traces at each temperature for the three radical SAM-based junctions, and Fig. 5b shows the Arrhenius plots for J at −1.0 V (see Supplementary Fig. 18 and Methods for temperature-dependent J (V) measurements of non-radical SAM-based junctions, that is, NRs). For the whole measured temperature range, the measured values of J (A cm −2 ) for the three radical SAMs are all temperature independent, which indicate the charge transport mechanism is in tunnelling regime. Figure 5: Temperature dependence measurements. ( a ) Semi-log plots of the average J (V) curves measured over the temperature range of 210–340 K at intervals of 10 K for Au TS -SC n PTM R SAMs with n =8, 10 and 12 and ( b ) Arrhenius plots of the average J at −1.0 V. The error bars represent the standard deviations of 10 J (V) curves. Full size image To investigate the dependence of J as a function of tunnelling distance ( d ), here we used carbon number n as the equivalent for d and plotted ‖ J ‖ > G (determined at −1.0 V) versus n ( Fig. 6 ). 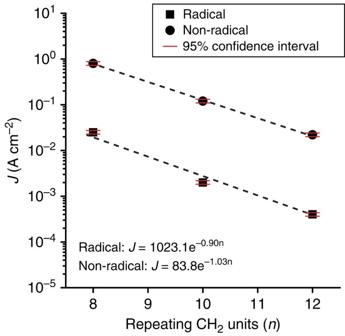Figure 6: General tunnelling equation fit. The average values ofJ(A cm−2) at −1.0 V as a function of carbon number (n) for AuTS-SCnPTMR/NR//GaOxcond/EGaIn junctions. The dashed lines represented the fits to the general tunnelling equation. The red error bars represent the 95% confidence interval. To this plot, we fitted the general tunnelling equation (equation (3)): Figure 6: General tunnelling equation fit. The average values of J (A cm −2 ) at −1.0 V as a function of carbon number ( n ) for Au TS -SC n PTM R/NR //GaO x cond /EGaIn junctions. The dashed lines represented the fits to the general tunnelling equation. The red error bars represent the 95% confidence interval. Full size image where β is the tunnelling decay coefficient (in n −1 ) and J 0 (A cm −2 ) is a constant including the contact resistance and it measures the current density flowing through the electrode-SAM interface in the hypothetical case of zero separation between the electrodes [52] . The values of β only show a small difference for both types of junctions ( β R =0.89±0.01 n −1 and a β NR =1.03±0.03 n −1 ) but the values of J 0 differ strongly in the magnitude (log J 0,R =3.0±0.2 and log J 0,NR =1.9±1.2). Here, the error bar represents the 95% confidence level from least absolute deviation (LAD) fitting (see procedure of LAD fitting in ref. 26 ). These β values are similar in value to those reported for insulating organic molecules ( n -alkanethiols), which have β values between 0.9 and 1.1 n −1 (refs 28 , 39 , 53 ). The magnitudes of the values of J 0 are in line with other SAM-based molecular junctions but at least 1,000 times lower than single molecular junctions due to the differences in effective contact area between the techniques [47] , [54] . It was reported before that the values of β are proportional to the square root of the δ E ME for coherent non-resonance tunnelling through a rectangular barrier, that is, (refs 55 , 56 ). The δ E ME values of PTM NR SAMs are consistently ∼ 2 times higher than PTM R SAMs, which leads to about a 1.4 times increase in β. This back of the envelope calculation is in line with our measured data that the β NR at −1.0 V is about 1.2 times higher than β R (this estimation does not take into account the shape of the barrier and the renormalization of the energy levels when bias is applied). This result also suggests that the decay rate is dominated by the length of the alkyl chain and the PTM moiety is effectively decoupled from the Au electrode by the long alkyl tether. This observation is supported by temperature-dependent measurements, which demonstrate that for over the entire measured temperature range, the values of J are independent of the temperature for the PTM R junctions. Along with the exponential decay of J with d , we believe that the mechanism of charge transport is direct tunnelling [53] , [57] . This interpretation also agrees with equation (2) and the large difference in J 0,R and J 0,NR values relates to the difference in δ E ME values: the radical SAM-based junctions have smaller δ E ME values and thus larger higher transmission probabilities ( T ) than the non-radical analogues. In previous reports some of us claimed that resonant tunnelling is important where the SOMO energy determines the tunnelling barrier height. These assumptions were based on electronic structure calculations using molecules in the gas phase without accounting for Fermi-level pinning as a result of the metal–thiolate bond. The energy level diagram shown in Fig. 1 is based on experimental data ( Table 1 ) from which we conclude that the empty levels define the tunnelling barrier height and not the filled levels. Although the exact shape of the tunnelling barrier inside the junctions during charge transport is not known, we believe that the energy-level diagram represents our system well considering the non-covalent nature of SAM//top contact. Although the junctions are asymmetric and the empty levels of the PTM R moieties are energetically and spatially very close to the Fermi level of the top-electrode and separated from the bottom electrode by the alkyl, we do not observe significant current rectification. In contrast, similar junctions but with Fc or bipyridyl (BIPY) end groups do rectify [26] , [58] . These diodes rectify currents because hopping (thermally activated charge transport) involving the Fc or BIPY is important. However, redox-active SAMs with p -quinone end groups resulted in rectifying EGaIn junctions with low rectification ratios of 3.5 (ref. 28 ). Although molecular asymmetry is needed to obtain rectification, the magnitude of rectification depends on many factors including the shape of the electrostatic potential profile [48] , the terminal group coupling with the EGaIn top electrode [48] , [58] or relaxation time of the charge carrier on the molecule (or activation energy for hopping) [16] , [59] . Currently, we do not know why certain end groups facilitate hopping while others do not. In summary, a family of PTM radical (which have single-occupied molecular orbitals), and the corresponding non-radical (which have filled molecular orbitals), derivatives of different molecular lengths bearing a thiol group has been synthesized and successfully integrated in molecular junctions of the type of Au TS -SC n PTM R/NR /GaO x cond /EGaIn. Temperature- and chain length-dependent measurements indicate that the mechanism of charge transport across all the junctions is direct tunnelling. This work exemplifies that stable free organic radicals are interesting systems, in addition to others, in molecular junctions because they have small SOMO/SUMO or HOMO/LUMO gaps. In addition, the possibility of having the radical and non-radical junctions make it possible to re-align the molecular energy levels with respect to the Fermi-levels of the metal contacts without altering the nature of the molecule—metal contacts or the backbone of the molecule and, thus, avoiding issues such as Fermi-level pinning. Our results demonstrate that intramolecular control over the energy-level alignment of molecular tunnelling junctions is a promising approach to control the electrical characteristics of two-terminal molecular junctions. We believe that in the future our findings may be extended to other types of junctions or to control, or perhaps induce, new electronic function. Synthesis The general procedure of the synthesis of PTM derivatives is outlined in Supplementary Fig. 1 . The detailed synthesis and characterization of PTM derivatives are described in the Supplementary Methods . The representative infrared (IR), cyclic voltammetry (CV), ultraviolet–visible and electron paramagnetic resonance (EPR) spectra of radicals are shown in Supplementary Figs 2–9 . Fabrication of template-stripped bottom-electrode We have reported before the procedure for template stripping using epoxy (EpoTek 353ND) [44] , [49] , [60] . Briefly, we deposited A 200-nm-thick Au (with a purity of 99.999% both from Super Conductor Materials Inc) film on clean Si(100) wafers by thermal deposition (Shen Yang Ke Yi, China). The evaporation rate was about 0.3 Å s −1 for the first 50 nm and then increased to ∼ 5 Å s −1 to deposit the remaining 150 nm and the deposition vacuum was about 2 × 10 −6 mbar. We cut the glass slides into pieces of 1 × 0.5 cm 2 and then cleaned them in a solution of H 2 SO 4 :H 2 O 2 =1:5 (in volume) at 80 °C for 20 min, and then washed with H 2 O to pH 7 and drying in a stream of N 2 gas. The glass slides were further cleaned by a plasma of air for 5 min at a pressure of 5 mbar. We dropped the epoxy on the Au surfaces and carefully added the glass slides on top of the epoxy. After the whole wafer was covered with glass slides, we cured the epoxy at 80 °C for 8 h in an oven (Epec). The final step was to lift off the glass slides with Au surfaces glued on them before immersion in the thiol solutions to minimize contamination of the Au TS surfaces by air. Formation of the SAMs Au TS surfaces were immersed in a freshly prepared solution of 0.5 mM of each compound in toluene (HPLC grade) for 24 h at 40 °C and then for an additional 24 h at room temperature. Always, before immersing the substrates, the solution was degassed with argon. During the SAM formation, the solution was kept in dark and under argon atmosphere to avoid the decomposition of the radical species. After the time indicated above, the substrates were removed from the solution and were washed with toluene and dichloromethane to remove any physisorbed materials. The modified substrates were characterized immediately after removal from the solution. The electrochemical characterization was performed using 300 nm Au evaporated on mica from Georg Albert (Germany). Before their use, the substrates were rinsed with acetone, dichloromethane and ethanol and then exposed to ozone for 20 min. Immediately after that the substrates were immersed in ethanol (HPLC grade) for at least 30 min. Before immersing the substrates in the PTM derivative solution, they were rinsed with ethanol and dried under nitrogen stream. Electrochemical characterization of the SAMs The three SAMs of Au-SC n PTM were electrochemically characterized by using CV performed with an AUTOLAB 204 with NOVA 1.9 software. We used a custom built electrochemical cell with a Pt-wire as counter electrode, Ag-wire as pseudo reference electrode and the modified Au(111) on mica as working electrode. The area exposed to the tetrabutylamonium hexafluorophosphate (TBAPF 6 ) in dichloromethane electrolyte solution (0.1 M) was 0.26 cm 2 . The CVs were recorded in the range +0.1 V to −0.6 V. The electrochemical measurements were performed in a Faraday cage. CV depicted in Supplementary Fig. 10 shows the CV of the R 10 SAM as representative for the different SAMs. Fabrication of PDMS top-electrodes We have reported the fabrication of the top-electrodes of Ga 2 O 3 /EGaIn stabilized in PDMS in detail elsewhere [51] . Since the fabrication methods are essentially the same, we only provide Supplementary Fig. 11 , which shows the microscope image of the through-hole filled with Ga 2 O 3 /EGaIn. A small gap of roughly 10 μm is present between the Ga 2 O 3 /EGaIn and the wall of the PDMS. In all the measurements reported here, we used electrodes with a geometrical contact area of about 7.1 × 10 2 μm. Fabrication of Au TS -SC n PTM R/NR //GaO x cond /EGaIn junctions The fabrication of the SAM-based junctions with cone-shaped tips of GaO x cond /EGaIn were reported previously [11] . Briefly, in our experiments we grounded the bottom electrode with a gold probe penetrating the SAMs and the top-electrode of GaO x cond /EGaIn was biased from 0 V→1.0 V→0 V→−1.0 V→0 V, with a step size of 50 mV and a delay of 0.1 s, to record the J (V) curves. The statistical analysis follows previous reported methods [11] and the results are listed in Table 1 . Stability measurement of Au TS -SC 8 PTM R/NR //GaO x cond /EGaIn junctions To investigate whether the junctions are stable and do not change during voltage cycling, we prepared junctions with the PDMS top-electrodes described in Methods section `Fabrication of PDMS top-electrodes' and measured 1,000 J (V) traces in the bias range of ±1.0 V. All the J (V) traces for both types of junctions (that is, with SAMs of R 8 (red) and NR 8 (black)) are plotted in Supplementary Fig. 12 . The shape of the J (V) traces did not change significantly and the values of J remained constant over 1,000 traces (plotted in Supplementary Fig. 12B for +1.0 V). Photoelectron spectroscopy We have reported the measurement procedures and analysis of synchrotron-based photoemission spectroscopy (PES) measurements (XPS and UPS) and NEXAFS spectroscopy at the SINS (Surface, Interface and Nanostructure Science) beamline of the Singapore Synchrotron Light Source (SSLS) elsewhere [54] . Briefly, the base pressure was kept at 1 × 10 −10 mbar. We used the Au 4 f 7/2 core level peak at 84.0 eV measured from a sputter-cleaned gold foil in electrical contact with the sample to calibrate the photon energy. We chose 350 eV for the Cl 2 p , S 2 p and C 1 s for the XPS measurements, and 60 eV for the valence band measurements. To measure the work function, we applied –10 V bias to the sample to overcome the work function of the analyser. All UPS spectra were referenced to the Fermi edge of Au and all PES spectra were normalized by the photon current. For NEXAFS, we measured the photon energy from 270 eV to 330 eV. Two take-off angles (90° and 40°) were used to probe the angle-dependence. We performed the least-square peak fit analysis with Voigt functions (Lorentzian (30%) and Gaussian (70%)) using XPSpeak software, and the sloping background was modelled using Shirley plus linear background correction [61] , [62] . Supplementary Figs 13–16 show the high-resolution PES spectra with fits of Cl 2 p , C 1 s and S 2 p of the SAMs of Au TS -SC n PTM R/NR at two different take-off angles 90° and 40°, respectively. Supplementary Fig. 17 shows the UPS and NEXAFS spectra of Au TS -SC n PTM NR ( n =8 and 10). The C 1 s high-resolution spectra show three components: (1) C–C single bond at ∼ 284.2 eV labelled C 1 , (2) the central C (αC) of the PTM moiety and the C=C group at ∼ 285.2 to ∼ 285.3 eV labelled C 2 , and (3) aromatic C–Cl at ∼ 286.4 eV labelled C 3 (ref. 62 ). The Cl 2 p spectra show typical doublet peaks. The doublet peak of the S 2 p spectra are solely (or mainly) contributed by the typical S–Au bond at the binding energy of 161.8 eV. The SAMs of R 8 and NR 8 show a small portion of low binding energy at ∼ 160.8 eV, which has been reported before and is assigned to chemical absorption of the SAMs at grain boundaries [62] . We summarized the fitting results of the XPS spectra of C 1 s and Cl 2 p in the form of the elemental ratio in Supplementary Table 2 . From Supplementary Table 2 , we can make three conclusions: (1) the decrease of C 1 /C 3 ratios from carbon number 8 to 12 indicate the SAMs are standing up; (2) the C 2 /C 3 ratios are constant at 90° emission but slightly decrease at 40° due to the attenuation of the first C connected to the PTM group and (3) the Cl/C 3 ratios are constant for different SAMs and the difference between 90° and 40° emission angle is caused by the large attention of the central C signal compared with the Cl atom. Determination of the surface coverage of the SAMs from the S 2 p spectra To calculate the surface coverage of the PTM R/NR SAMs, we determined the integrated intensity of Cl 2 p spectra ( I Cl ) of the PTM R/NR and S(CH 2 ) 10 CH 2 Cl (SC 11 Cl) SAMs (listed in the Supplementary Table 1 ). Since the Cl atoms were connected to the terminal groups of the SAMs, the I Cl can be related to the surface coverage of the SAMs. The relative surface coverage was calculated by comparing the I Cl of the PTM R/NR SAMs, which divided by 14 (PTM R/NR SAMs contains 14 Cl atoms), against that of SC 11 Cl SAMs. The surface coverage of SC 11 Cl SAMs on Ag has been reported before and is 1.1 × 10 −9 mol cm −2 (ref. 29 ). Thus, we compared the values of I Cl of the PTM R/NR SAMs against those of the SC 11 Cl SAMs to calculate the relative surface coverage of the PTM R/NR SAMs ( Supplementary Table 1 ). We estimated the uncertainties to be about 5% from the fitting errors of Cl 2 p spectra. However, we note that not all of the 14 Cl atoms on the PTM moiety are located at the top of the SAMs, and the signal of at least 4 Cl atoms (connected to the phenyl ring with alkyl chain) are attenuated by half of the length ( ∼ 6.3 Å) of the PTM moiety. Thus, the surface coverage calculated by XPS here was underestimated by at least 13% (= ). Nevertheless, the relative surface coverages are the same for all the PTM SAMs which support our conclusion that we did not change the supramolecular structure of the PTM R/NR SAMs. We also estimated the theoretical surface coverage of these SAMs formed on the Au(111) surface, and the dimension of the PTM moiety was calculated from CPK model. Since the PTM moiety is a planer-triangle, its projection on the x–y plane changes between rectangles (or a parallelogram dependent on the molecular tilt angle which we do not know). We estimated a surface coverage of 1.8 × 10 −10 mol cm −2 from the simple case of rectangle projection (side lengths: a =12.6 Å and b =7.4 Å). The surface coverage estimated from XPS is similar to the theoretical estimation. Determination of the thickness of the SAMs from the S 2 p spectra We have reported the methods to fit the spectra and to calculate the SAM thickness from angle-dependent XPS measurements in ref. 48 . We only give a short description here. The SAM thickness ( d , nm) can be expressed as the sum of the Au–S bond ( d Au–S =1.8 Å) [63] and the over layer thickness (the distance from the middle of the S atom to vacuum) d 2 in equation (4) The different angles of the incident light ( γ ) result in different emission area on the samples. To normalize the footprint of incident light, we calculate the effective intensity ( I θ ) where I is the integrated intensity of the peak. The values of I θ are exponentially dependent on d 2 and on the take-off angle where the d 1 (=1.5 Å) is estimated from the radius of S atoms and the S–C bond, and λ (=8 Å) is the inelastic mean free path [62] . We can rewrite the equation (6) to calculate the value of d 2 The S 2 p spectra along with fits are shown in Supplementary Figs 12–15 , and the results are listed in Supplementary Table 3 . The uncertainty of ±2 Å takes into account the fitting errors and the angular misalignment due to sample mounting. Calculation of LUMO energy level from NEXAFS spectra We determined the SUMO or LUMO level with respect to the Fermi level of the electrode by the binding energy of the C 1 s core level of the PTM from the XPS spectra ( Supplementary Figs 13–18 ) and the SUMO or LUMO peak from the NEXAFS spectra with a correction of 0.5 eV for core–hole exciton-binding energy to take into account the core–hole attraction effect. Others have reported correction factors in the range of 0.1–2.0 eV (ref. 64 ), but we have used 0.5 eV also for other types of SAMs as described in the supporting information of ref. 60 . Since we used for both types of junctions with NR and R SAMs the same correction factor, the energy levels for both types of junctions would shift equally in case one would chose different correction factors and hence will not affect our conclusions. Temperature-dependent measurement of a junction with a SAM of NR 8 We used EGaIn top-electrodes stabilized in a through-hole in PDMS to form stable junctions, and measured the temperature-dependent J (V) in a probe station as mentioned in the main text. Supplementary Fig. 18 shows the J (V) traces recorded at 250–330 K at intervals of 10 K. Both the Arrhenius plots and the J (V) traces show that the junction characteristics are independent of temperature as expected, since the non-radical SAMs have larger molecular energy gaps than their radical counterparts and behave as tunnelling barrier. LAD fitting As mentioned in the manuscript, we performed LAD fitting of the tunnelling equation (equation (3) in the main text) to the full data set of log 10 | J | at different applied bias ( V ) from −1.0 V to −0.1 V. The details of the LAD fitting have been reported in ref. 65 . Supplementary Fig. 19 shows the plot of the tunnelling decay coefficient ( β ) against V . We found that the value of β of the junctions with SAMs of PTM NR is consistently ∼ 1.2 times higher than that of PTM R . Data availability The data that support the findings of this study are available from the corresponding author upon request. How to cite this article: Yuan, L. et al . Chemical control over the energy-level alignment in a two-terminal junction. Nat. Commun. 7:12066 doi: 10.1038/ncomms12066 (2016).